TRPV4 disrupts mitochondrial transport and causes axonal degeneration via a CaMKII-dependent elevation of intracellular Ca2+ 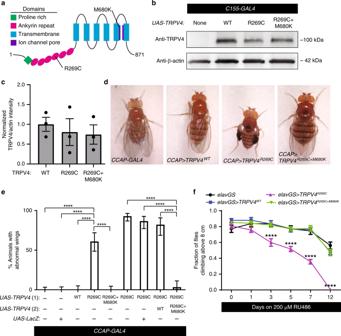Fig. 1: A neuropathy-causing TRPV4 variant causes channel pore-dependent neuronal dysfunction inDrosophila. aSchematic of TRPV4 domain structure with neuropathy-causing (R269C) and pore-inactivating (M680K) mutations indicated.bRepresentative western blot of protein lysates from the heads of adultDrosophilaexpressing TRPV4(mod) variants under the control ofC155-GAL4.cNormalized mean ± SEM band intensities from three independent western blots. One-way ANOVA (p= 0.778).dImages of flies expressing no TRPV4, TRPV4WT(mod), TRPV4R269C(mod), and TRPV4R269C+M680K(mod) in NCCAP.ePercentage ± 95% CI of flies with unexpanded wings ind. From left to rightn= 115, 102, 73, 64, 82, 114, 75, 45, and 61 flies.Χ2of all groups (p< 0.0001) followed by pairwise two-sided Fisher’s exact test.fClimbing performance of flies inducibly expressing TRPV4 (high) variants. Flies induced at 1–3 days post eclosion with 200 μM RU486. Mean ± SEM.n= 10 vials of 10 flies per genotype. Two-way ANOVA (p< 0.0001), Tukey’s post hoc test, asterisks indicate difference from all other genotypes. For all panels: ****p< 0.0001. The cation channel transient receptor potential vanilloid 4 (TRPV4) is one of the few identified ion channels that can directly cause inherited neurodegeneration syndromes, but the molecular mechanisms are unknown. Here, we show that in vivo expression of a neuropathy-causing TRPV4 mutant (TRPV4 R269C ) causes dose-dependent neuronal dysfunction and axonal degeneration, which are rescued by genetic or pharmacological blockade of TRPV4 channel activity. TRPV4 R269C triggers increased intracellular Ca 2+ through a Ca 2+ /calmodulin-dependent protein kinase II (CaMKII)-mediated mechanism, and CaMKII inhibition prevents both increased intracellular Ca 2+ and neurotoxicity in Drosophila and cultured primary mouse neurons. Importantly, TRPV4 activity impairs axonal mitochondrial transport, and TRPV4-mediated neurotoxicity is modulated by the Ca 2+ -binding mitochondrial GTPase Miro. Our data highlight an integral role for CaMKII in neuronal TRPV4-associated Ca 2+ responses, the importance of tightly regulated Ca 2+ dynamics for mitochondrial axonal transport, and the therapeutic promise of TRPV4 antagonists for patients with TRPV4-related neurodegenerative diseases. Congenital distal spinal muscular atrophy (CDSMA), scapuloperoneal spinal muscular atrophy (SPSMA), and Charcot-Marie-Tooth disease type 2C (CMT2C) are inherited degenerative diseases of the peripheral nervous system caused by mutations in the gene encoding the transient receptor potential vanilloid 4 (TRPV4) cation channel [1] , [2] , [3] . Peripheral nerve degeneration in these disorders results in muscle weakness, particularly of limb, diaphragm, and vocal fold muscles, the latter of which can be life threatening. They are strikingly variable in severity, ranging from severe, congenital onset to mild, late adult onset. The mutations are dominantly inherited missense mutations and each is capable of causing a wide spectrum of disease severities even within the same family. TRPV4 is a cell surface-expressed, non-selective cation channel that is preferentially permeable to Ca 2+ and is activated by mechanical, osmotic, and chemical stimuli [4] . The majority of neuropathogenic mutations are present in the intracellular amino-terminal ankyrin repeat domain [1] , [2] , [3] , [5] , [6] , where it has been postulated that they may alter inter- or intra-protein–protein interactions. The consequences of mutations of TRPV4 have been studied in cultured cells with conflicting results. Some studies suggest that neuropathy-causing mutations lead to a gain of TRPV4 ion channel function [1] , [2] , [5] , [6] , whereas others argue they cause a loss of function [3] . No studies have yet examined the effects of neuropathy-causing TRPV4 mutations on neurons in vivo. Establishing the pathogenic mechanisms of TRPV4 mutations has particular relevance for therapeutics development, as small molecule TRPV4 antagonists have proven safe in human clinical trials [7] and could be repurposed for neurological disease indications. There are very few examples of ion channels that are directly implicated in the process of neurodegeneration, as most neurological disease-associated channelopathies are paroxysmal disorders such as epilepsy or migraine [8] . Investigating how TRPV4 mutations cause peripheral neuropathy provides an opportunity to understand the molecular events linking an ion channel and Ca 2+ homeostasis to the process of neurodegeneration. Although Ca 2+ homeostasis is dysregulated in many neurodegenerative disorders, it is unknown whether Ca 2+ dysregulation is a primary or secondary pathological event. Ca 2+ regulates both the initiation of fast axonal transport as well as sustained transport of cargos along axons [9] , [10] , and disruptions of axonal transport are implicated in many neurodegenerative diseases, particularly peripheral nerve disease [11] , [12] . Several forms of hereditary neuropathy are caused by mutations in genes encoding proteins that regulate axonal transport such as kinesin ( KIF5A ), dynein ( DYNC1H1 ), and neurofilament ( NEFL ) [12] . Moreover, the most common form of axonal CMT is caused by mutations of mitofusin 2 ( MFN2 ), which are associated with impaired axonal transport of mitochondria [13] , [14] , [15] . Interrogation of the cellular events underlying TRPV4-associated neuropathy may provide insights into mechanistic links between Ca 2+ and impaired axonal transport in neurodegenerative disease. In this study, we explored the consequences of mutant TRPV4 expression in Drosophila and cultured primary mammalian neurons. We show that mutant TRPV4 causes neuronal dysfunction and degeneration that are dependent on TRPV4 channel activity. Using an unbiased forward genetic screen in Drosophila , we found that TRPV4-mediated increases in intracellular Ca 2+ require CaMKII, revealing a central role for CaMKII in TRPV4-associated axonal degeneration. Moreover, we observe axonal mitochondrial transport defects downstream of TRPV4 channel activation. Our data suggest that neuropathogenic TRPV4 mutations sensitize the TRPV4 ion channel resulting in CaMKII-dependent Ca 2+ entry that both disrupts mitochondrial axon transport and causes axonal degeneration. TRPV4 mutations disrupt neuron function via the TRPV4 pore Human TRPV channel expression rescues phenotypes resulting from loss-of-function mutations in Drosophila TRPV channels, demonstrating functional conservation across species [16] . To evaluate neuropathogenic TRPV4 mutations in vivo, we generated transgenic Drosophila lines that express human TRPV4 under the control of the GAL4/UAS binary expression system. We primarily utilized three TRPV4 variants in our studies: wild type TRPV4 (TRPV4 WT ), a neuropathy-causing mutant (TRPV4 R269C ), and TRPV4 R269C with a second engineered mutation known to block the TRPV4 ion-conducting pore (TRPV4 R269C+M680K ) (Fig. 1a ) [1] . We identified low-, moderate-, and high-expressing transgenic lines (TRPV4(low), TRPV4(mod), and TRPV4(high)) in which these three variants are expressed at similar levels (Fig. 1b, c , Supplementary Fig. 1a, b ). When expressed in all neurons using the C155-GAL4 driver, flies expressing TRPV4 R269C , but not TRPV4 WT or TRPV4 R269C+M680K , fail to appropriately expand their wings after eclosion (Supplementary Fig. 1c ). This phenotype is dose-dependent, as high-level expression of TRPV4 R269C markedly increases the penetrance of the wing phenotype (Supplementary Fig. 1c ). A second neuropathy-causing mutant (TRPV4 R232C ) also causes this wing expansion phenotype (Supplementary Fig. 1c ), suggesting that this phenotype is common to neuropathy-associated variants. Fig. 1: A neuropathy-causing TRPV4 variant causes channel pore-dependent neuronal dysfunction in Drosophila . a Schematic of TRPV4 domain structure with neuropathy-causing (R269C) and pore-inactivating (M680K) mutations indicated. b Representative western blot of protein lysates from the heads of adult Drosophila expressing TRPV4(mod) variants under the control of C155 - GAL4 . c Normalized mean ± SEM band intensities from three independent western blots. One-way ANOVA ( p = 0.778). d Images of flies expressing no TRPV4, TRPV4 WT (mod), TRPV4 R269C (mod), and TRPV4 R269C+M680K (mod) in N CCAP . e Percentage ± 95% CI of flies with unexpanded wings in d . From left to right n = 115, 102, 73, 64, 82, 114, 75, 45, and 61 flies. Χ 2 of all groups ( p < 0.0001) followed by pairwise two-sided Fisher’s exact test. f Climbing performance of flies inducibly expressing TRPV4 (high) variants. Flies induced at 1–3 days post eclosion with 200 μM RU486. Mean ± SEM. n = 10 vials of 10 flies per genotype. Two-way ANOVA ( p < 0.0001), Tukey’s post hoc test, asterisks indicate difference from all other genotypes. For all panels: **** p < 0.0001. Full size image Drosophila wing expansion is controlled by crustacean cardioactive peptide-expressing neurons (N CCAP ), which initiate motor programs upon eclosion that drive wing expansion [17] , [18] . Selective expression of TRPV4 R269C (mod) in these neurons using CCAP-GAL4 recapitulates the unexpanded wing phenotype observed with pan-neuronal expression (Fig. 1d, e ). Flies expressing TRPV4 R269C+M680K have no wing phenotype, even with high-level pan-neuronal expression (Fig. 1d, e , Supplementary Fig. 1c ). Furthermore, co-expression of TRPV4 R269C+M680K (mod) strongly suppresses the phenotype caused by TRPV4 R269C (mod), suggesting that the pore-inactivating mutation blocks channel function both in cis and in trans (Fig. 1e ), consistent with the known tetrameric structure of TRPV4 ion channels [19] . TRPV4 mutations are associated with congenital onset disease in humans, but also with later onset, slowly progressive symptoms. To assess whether mutant TRPV4 can cause progressive disease after adult development, we utilized an inducible pan-neuronal GAL4 driver elav - GeneSwitch ( elavGS ) [20] to express TRPV4(high) variants in early adulthood. Flies induced to express TRPV4 R269C (high) by feeding with RU486 show a marked, progressive decline in climbing performance and are unable to climb 12 days after induction of expression (Fig. 1f ). In contrast, flies expressing either TRPV4 WT (high) or TRPV4 R269C+M680K (high) show no difference in climbing performance compared with flies carrying elavGS alone (Fig. 1f ). Together, these data demonstrate that TRPV4 R269C expression can cause both early- and late-onset neuronal dysfunction in vivo, and that this neurotoxicity requires a functional ion channel pore. TRPV4 R269C causes axonal and dendritic degeneration Degeneration and loss of peripheral nerve axons are characteristic pathological features of CMT [21] . To test whether TRPV4 R269C causes neuronal degeneration, we assessed class IV larval dendritic arborization (C4da) neurons, sensory neurons with dendrites that tile the Drosophila larval body wall [22] , in wandering third instar larvae using ppk-GAL4 [23] . We selected these neurons for functional and morphological analysis owing to their genetic tractability, experimental accessibility, and their previous use in a Drosophila model of CMT [24] . As compared with control flies expressing TRPV4 WT (high), TRPV4 R269C+M680K (high), or no TRPV4, flies expressing TRPV4 R269C (high) show a marked loss of C4da neuron axonal projections into the ventral nerve cord (Fig. 2a, b ) and severely reduced dendritic arborizations within the body wall (Fig. 2c, d ). These phenotypes are not observed with overexpression of other cation channels previously shown to activate or silence Drosophila neurons and disrupt N CCAP function [18] , [25] (Supplementary Fig. 2a, c ), suggesting these axonal and dendritic degeneration phenotypes are not caused by altered neuronal activity. Fig. 2: High TRPV4 R 269C expression disrupts C4da neuron axonal and dendritic projections. Confocal projections of C4da neuron axonal projections a and dendrites c from wandering third instar larvae expressing TRPV4 (high) variants. b Mean ± SEM normalized projection areas in a . n = 9 (control), 9 (TRPV4 WT ), 10 (TRPV4 R269C ), and 9 (TRPV4 R269C+M680K ) larvae. Two-way ANOVA ( p < 0.0001), Tukey’s post hoc test. d Sholl analysis of neurons in c . Mean ± SEM. n = 5 cells, one per larva, from five larvae per genotype. Asterisks denote difference from no TRPV4 (control). Two-way ANOVA ( p < 0.0001), Tukey’s post hoc test. Confocal stacks of axonal projections e and dendrites f of flies expressing TRPV4 R269C (high) raised on food with either DMSO or 100 μM GSK219. g Sholl analysis of dendritic phenotypes in f . Control from d shown for reference. Mean ± SEM. n = 6 cells from three larvae for DMSO, n = 10 cells from five larvae for GSK219. Asterisks denote differences from DMSO. Two-way ANOVA ( p < 0.0001), Tukey’s post hoc test. Scale bar, 25 µm in a and e and 50 µm in c and f . For all panels: * p < 0.05, ** p < 0.01, *** p < 0.001, and **** p < 0.0001. Full size image To determine whether the morphological changes in C4da neurons are owing to degeneration or impaired development, we imaged C4da neuron axonal projections and dendrites in larvae at 96 hours (late second instar) and 120 hours (early third instar) after egg laying (AEL). At 96 hours AEL, we observe no significant differences in either axonal projections or number of dendritic branches (Supplementary Fig. 3a, c ). However, at 120 hours AEL, we observe axonal swellings (Supplementary Fig. 3a , 2× zoom, green arrows), fragmentation of distal axonal projections (Supplementary Fig. 3a , 2× zoom, magenta arrow), and a reduction of dendritic branching (Supplementary Fig. 3b, c ) in larvae expressing TRPV4 R269C (high). Like the phenotypes in N CCAP , axonal degeneration in C4da neurons is TRPV4-dosage dependent, as moderate expression of TRPV4 R269C does not alter axonal projection area (Supplementary Fig. 3d, e ). Of note, high expression (but not moderate expression) of TRPV4 WT causes a mild wing expansion phenotype and a mild loss of axonal projections and dendritic branching (Supplementary Fig. 1c , Fig. 2a, b ). Thus, TRPV4 R269C causes neurodegeneration in vivo in a dose-dependent manner, and sufficient expression of TRPV4 WT can cause similar, yet more mild, phenotypes. These observations are consistent with a gain-of-TRPV4 function mechanism of toxicity caused by the R269C mutation. TRPV4 antagonists suppress TRPV4-mediated neurodegeneration As genetic inactivation of the TRPV4 R269C channel pore rescues neurotoxicity (Figs. 1 d, f, 2a, d , and Supplementary Fig. 1c ), we next asked if TRPV4 could be blocked pharmacologically to suppress the axonal and dendritic phenotypes mediated by TRPV4 R269C (high). We tested the selective TRPV4 antagonist GSK2193874 (GSK219) because TRPV4 antagonists are in clinical development for the treatment of pulmonary edema during heart failure [7] , [26] . Embryos expressing TRPV4 R269C were raised on food containing either GSK219 or DMSO vehicle alone throughout larval development. Remarkably, GSK219 treatment of TRPV4 R269C (high) flies reduces axonal degeneration and dendritic branching defects as compared to vehicle treatment alone (Fig. 2e, g ). CaMKII is required for TRPV4 R269C -mediated neurotoxicity To identify genes that contribute to TRPV4 R269C -mediated neurotoxicity, we performed RNAi- and overexpression-based screens for genetic modifiers of the wing expansion phenotype caused by moderate TRPV4 R269C expression in N CCAP . With the goal of identifying potential therapeutic targets, we specifically screened genes that are conserved in humans, potentially druggable [27] , and expressed in the Drosophila nervous system (flybase.org). We also screened fly orthologues of genes previously implicated in CMT. In total, we evaluated 692 transgenic lines covering 502 genes and identified 8 genes that reduce the penetrance of the TRPV4 R269C -mediated wing phenotype to <25% compared with the 70–100% penetrance observed in control flies (Fig. 3a , Supplementary Data 1 ). Fig. 3: CaMKII is required for TRPV4 R269C -mediated neuronal toxicity. a Histogram of results from genetic modifier screen against TRPV4 R269C toxicity in N CCAP . Dashed magenta lines denote upper and lower bounds of control lines. b Images of flies expressing TRPV4 R269C (mod) ± CaMKII RNAi. c Percentage ± 95% CI of flies with unexpanded wings when co-expressing TRPV4 R269C (mod) and different CaMKII RNAi fly lines. A = TRiP collection lines, B = Vienna GD collection lines, and C = Vienna KK collection lines. From left to right n = 65, 59, 60, 25, 65, 66, and 90 flies. Χ 2 test of all groups ( p < 0.0001) followed by pairwise two-sided Fisher’s exact test. d Confocal stacks of axonal projections in C4da neurons expressing TRPV4 R269C (high) ± CaMKII RNAi. e Mean ± SEM innervation in d . n = 5, 4, and 5 larvae, respectively. One-way ANOVA ( p < 0.0002), Tukey’s post hoc test. Scale bar, 25 µm. f Climbing performance of flies 7 days after induction of expression of TRPV4 R269C (high) ± CaMKII RNAi with 200 μM RU486. Mean ± SEM. n = 10 vials of 10 flies per genotype. Two-way ANOVA ( p < 0.0001), Tukey’s post hoc test. g Percentage ± 95% CI of flies with unexpanded wings when co-expressing TRPV4 R269C (low) with variants of CaMKII. T287D 1 and T287D 2 denote independent UAS - CaMKII T287D lines. From left to right n = 63, 55, 68, 44, 23, 33, 28, 23, 2, and 3 flies. Χ 2 test of all groups ( p < 0.0001) followed by pairwise two-sided Fisher’s exact test. For all panels: ** p < 0.01, **** p < 0.0001. Full size image The most potent genetic modifier identified in this screen was Ca 2+ /calmodulin-dependent protein kinase II (CaMKII), a key regulatory kinase of many neuronal signaling pathways [28] . Knockdown of the single Drosophila CaMKII using four independent RNAi lines on three distinct genetic backgrounds reduces the penetrance of the TRPV4 R269C -mediated wing phenotype to 0–10% (Fig. 3a, c ). CaMKII knockdown is also sufficient to ameliorate other TRPV4 R269C -mediated phenotypes including the loss of C4da neuron axonal projections in flies expressing TRPV4 R269C (high) (Fig. 3d, e ) and the climbing phenotype at 7 days post induction of elavGS (Fig. 3f ). To test whether CaMKII overexpression can enhance TRPV4 R269C -mediated neurotoxicity, we generated a UAS line that expresses TRPV4 R269C at very low levels via site-directed insertion (TRPV4 R269C (low)) [29] . Although overexpression of either TRPV4 R269C (low) or CaMKII alone in N CCAP did not impair wing expansion, simultaneous overexpression of both CaMKII and TRPV4 R269C (low) causes a highly penetrant wing phenotype (Fig. 3g ). Upon binding Ca 2+ , CaMKII is autophosphorylated at T287 enabling Ca 2+ -independent, constitutive CaMKII activity [28] . Interestingly, in the absence of TRPV4 R269C , expression of the constitutively active T287D phosphomimetic mutant of CaMKII [30] , but not the Ca 2+ -dependent T287A mutant, cause a highly penetrant wing phenotype (Fig. 3g ). These data suggest that CaMKII autophosphorylation is necessary and sufficient to mediate neurotoxicity caused by TRPV4 R269C . A secondary genetic screen examining known CaMKII target proteins and pathways did not identify individual modifiers that similarly rescued TRPV4 R269C -mediated toxicity, suggesting that either multiple CaMKII substrates are involved or that CaMKII is working through an unknown substrate (Supplementary Data 2 ). TRPV4 R269C causes CaMKII-dependent hyperexcitability N CCAP regulate Drosophila wing expansion in a manner that is sensitive to changes in excitability [17] , [18] . To test whether TRPV4 ion channel activity influences the excitability of N CCAP , we utilized whole-cell perforated patch-clamp recording [25] , [31] to measure the activity of N CCAP in flies expressing TRPV4 WT (mod), or TRPV4 R269C (mod). A tracer dye was injected into the neurons following recording to validate cell identity (Supplementary Fig. 4 ). Expression of TRPV4 R269C (mod) increases the spontaneous mean firing rate of N CCAP by 5.8-fold, compared with an approximately twofold increase brought about by TRPV4 WT (mod) expression (Fig. 4a, b ). In addition, TRPV4 R269C (mod) increases the intrinsic excitability of N CCAP as measured by the mean firing rate in response to injected current (Supplementary Fig. 5a ). We observe no change in the mean resting membrane potential (RMP) (Supplementary Fig. 5b ), but subthreshold membrane potential variability (Δ ramp), a property that may allow neurons to reach threshold more frequently, is increased in flies expressing TRPV4 R269C (mod) (Supplementary Fig. 5c ). Fig. 4: TRPV4 R269C mediates a reversible, Ca 2+ - and CaMKII-dependent increase in neuronal excitability. a Traces of N CCAP spontaneous activity in flies expressing no TRPV4, TRPV4 WT (mod), or TRPV4 R269C (mod) ± 5 mM BAPTA. b Mean firing rates from a . Mean ± SEM. n = 9 (no TRPV4), 8 (TRPV4 WT ), 9 (TRPV4 R269C ), 5 (no TRPV4 + BAPTA), 5 (TRPV4 WT + BAPTA), and 6 (TRPV4 R269C + BAPTA) flies. Two-way ANOVA ( p = 0.0017), Tukey’s post hoc test. c Mean firing rate after incubation with GSK219. Mean ± SEM. TRPV4 WT n = 8, 6, and 4 flies for 0, 100, and 500 nM TRPV4 R269C n = 8, 5, 8, and 4 flies for 0, 100, 500, and 10,000 nM. 0 nM values are the same as shown in b . One-way ANOVA ( p < 0.0001 (TRPV4 WT ), p = 0.0169 (TRPV4 R269C )), Tukey’s post hoc test. d Traces of N CCAP spontaneous activity in flies expressing TRPV4 R269C ± CaMKII RNAi . e Mean firing rate in d . Mean ± SEM. n = 6 per genotype. Unpaired two-tailed t test. p = 0.0017. For all panels: * p < 0.05, ** p < 0.01, *** p < 0.001, **** p < 0.0001. Full size image To test whether changes in excitability are related to changes in Ca 2+ , we applied the cell-permeant Ca 2+ chelator 1,2-bis( O -aminophenoxy)ethane- N,N,N’,N’ -tetraacetic acid (BAPTA). BAPTA application blocks the increased spontaneous mean firing rate (Fig. 4a, b ), intrinsic N CCAP excitability (Supplementary Fig. 5d ) and Δ ramp (Supplementary Fig. 5f ) caused by TRPV4 WT (mod) and TRPV4 R269C (mod). Similarly, the TRPV4-selective antagonist GSK219 also reduces spontaneous activity (Fig. 4c ), intrinsic excitability (Supplementary Fig. 5g ), and Δ ramp (Supplementary Fig. 5i ) in a dose-dependent fashion, as does knockdown of CaMKII (Fig. 4d, e , Supplementary Fig. 6a, c ). Collectively, these data demonstrate that reversible alterations of TRPV4 R269C -mediated excitability are dependent on both intracellular Ca 2+ and CaMKII. TRPV4 R269C has enhanced response to agonist stimulation To evaluate if TRPV4 activity alters intracellular Ca 2+ dynamics in neurons in vivo, we co-expressed the genetically encoded calcium indicator GCaMP6s [23] with TRPV4(mod) variants in C4da neurons. We analyzed Ca 2+ dynamics by measuring changes in GCaMP6s fluorescence intensity in C4da neuronal somata of dissected third instar larvae after administration of vehicle or the TRPV4-selective agonist GSK1016790A (GSK101) [32] , [33] . C4da neurons expressing TRPV4 R269C (mod) demonstrate a faster Ca 2+ response upon GSK101 application than C4da neurons expressing TRPV4 WT (mod), with a time to half maximum intensity ( t 1/2 max ) of 22 ± 2.4 s (best fit parameter ± SEM) for TRPV4 R269C compared with a t 1/2 max of 41 ± 3.0 s for TRPV4 WT ( p < 0.0001) (Fig. 5a, b ). There is also a trend toward a higher maximum response in TRPV4 R269C -expressing larvae (Fig. 5a, b ). Control C4da neurons expressing no TRPV4 or TRPV4 R269C+M680K show no change in Ca 2+ levels in response to GSK101, and no neurons responded to DMSO treatment alone (Fig. 5a, b , Supplementary Fig. 7a ). We also monitored spontaneous calcium transients in the larval ventral nerve cord using myristoylated GCaMP5 in C4da neurons expressing TRPV4 variants. Notably, C4da neurons expressing TRPV4 R269C (mod) have a marked increase in spontaneous calcium transients in axonal projections compared with control neurons and neurons expressing TRPV4 WT (Supplementary Fig. 7b and Supplementary Videos 1 – 3 ). This increase is abolished by inclusion of the M680K mutation (Supplementary Fig. 7b and Supplemental Video 4 ), suggesting that the increase in calcium transient frequency is TRPV4 channel pore-dependent. Fig. 5: The R269C mutation enhances TRPV4-mediated Ca 2+ influx in fly and mouse neurons. a Confocal images of GCaMP6s in larval C4da neurons expressing the indicated transgenes before and 180 s after application of 40 nM GSK101 at t = 0 s. Scale bar, 50 μm. b Change in somal GCaMP6s fluorescence over baseline (ΔF/F) of the genotypes shown in a . Mean ± SEM. n = 8 (no TRPV4), 8 (TRPV4 WT ), 7 (TRPV4 R269C ) and 10 (TRPV4 R269C+M680K ). Non-linear regression (dashed lines, logistic model) indicates TRPV4 WT t 1/2max = 41 ± 3.0 s was greater than TRPV4 R269C t 1/2max = 22 ± 2.4 s ( p < 0.0001, unpaired two-tailed t test). Maximum response 0.91 (TRPV4 R269C ) and 0.73 (TRPV4 WT ) ( p = 0.06, unpaired two-tailed t test) c Images of the Fura-2AM ratio in primary mouse trigeminal neurons transduced with TRPV4 WT or TRPV4 R269C before and after the application of 30 nM GSK101. Scale bar, 50 μm. d Mean ± SEM Fura-2AM ratio over time of the images in c . Drug added at t = 0. n = 44 (TRPV4 WT ) and 48 (TRPV4 R269C ) neurons from 12 wells per genotype from three separate preparations. Non-linear regression (dashed lines, logistic model) indicates TRPV4 WT t 1/2max = 28 ± 8.5 s and TRPV4 R269C t 1/2max = 16 ± 3.8 s ( p = 0.2, unpaired two-tailed t test). Maximum responses TRPV4 WT = 0.9, TRPV4 R269C = 1.2 ( p < 0.0001, unpaired two-tailed t test). e Mean ± SEM Fura-2AM ratio over time in response to 30 nM GSK101 at t = 0 in neurons expressing TRPV4 WT and pre-treated for 4 hours with 10 μM KN-93 or KN-92, n = 44 (KN-92) and 28 neurons (KN-93) from 12 wells per genotype from three separate preparations. Two-way ANOVA, Geisser-Greenhouse correction ( p < 0.0001), Tukey’s post hoc test. For all panels: * p < 0.05,** p < 0.01, *** p < 0.001. Full size image To determine whether similar effects are observed in mammalian neurons, we cultured primary mouse trigeminal neurons and transduced them with equivalent titers of lentiviral vectors encoding TRPV4 WT -EGFP or TRPV4 R269C -EGFP (Supplementary Fig. 8a, b ). Both TRPV4 WT -EGFP and TRPV4 R269C -EGFP express at equivalent levels and localize to the cell cortex in the somata and neurites (Supplementary Fig. 8c, d ). We determined somal Ca 2+ signals by measuring the Fura-2AM 340/380 ratio. As predicted based on calcium imaging of nonneuronal cells [5] , there is a small but statistically significant increase in baseline calcium levels in neurons expressing TRPV4 R269C compared with TRPV4 WT (Supplementary Fig. 8e ). Like fly neurons, mouse trigeminal neurons transduced with TRPV4 R269C -EGFP respond more rapidly and more robustly to GSK101 with a t 1/2 max of 16 ± 3.8 s (best fit parameter ± SEM) as compared with TRPV4 WT (28 ± 8.5 s) (Fig. 5c, d ). The maximum response of TRPV4 R269C (1.2 ± 0.016) is greater than that of TRPV4 WT (0.91 ± 0.014) ( p < 0.0001). Collectively, these data indicate that the R269C mutation sensitizes the TRPV4 channel in Drosophila neurons in vivo and primary mammalian neurons in vitro, consistent with the gain-of-ion channel function phenotypes observed in flies. To determine whether CaMKII is required for TRPV4-induced Ca 2+ influx, we treated primary trigeminal neurons expressing TRPV4 WT -EGFP with the calmodulin-targeting CaMKII inhibitor KN-93 or its inactive analog KN-92 [34] , [35] . Remarkably, KN-93 significantly attenuates Ca 2+ responses to GSK101 in neurons expressing TRPV4 WT -EGFP, whereas those treated with KN-92 respond normally to agonist stimulation (Fig. 5e ). We observe similar inhibitory effects when treating with autocamtide-2-related inhibitory peptide (AIP), a small peptide CaMKII inhibitor [36] (Supplementary Fig. 9a ). The effect of CaMKII inhibition is not owing to altered TRPV4 surface expression, as CaMKII inhibition does not alter the cortical localization of TRPV4-EGFP (Supplementary Fig. 9b, e ). Furthermore, CaMKII inhibition with KN-93 also prevents increases of intracellular Ca 2+ levels mediated by endogenous TRPV4 in an immortalized rat dorsal root ganglion cell line [37] (Supplementary Fig. 10a, c ). These data indicate that CaMKII is required for TRPV4-mediated increases in intraneuronal Ca 2+ levels. TRPV4 R269C disrupts mitochondrial axon transport Axonal transport of mitochondria is regulated by intracellular Ca 2+ [9] , [10] , [38] . 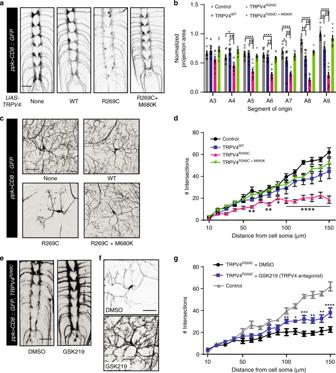Fig. 2: High TRPV4R269Cexpression disrupts C4da neuron axonal and dendritic projections. Confocal projections of C4da neuron axonal projectionsaand dendritescfrom wandering third instar larvae expressing TRPV4 (high) variants.bMean ± SEM normalized projection areas ina.n= 9 (control), 9 (TRPV4WT), 10 (TRPV4R269C), and 9 (TRPV4R269C+M680K) larvae. Two-way ANOVA (p< 0.0001), Tukey’s post hoc test.dSholl analysis of neurons inc. Mean ± SEM.n= 5 cells, one per larva, from five larvae per genotype. Asterisks denote difference from no TRPV4 (control). Two-way ANOVA (p< 0.0001), Tukey’s post hoc test. Confocal stacks of axonal projectionseand dendritesfof flies expressing TRPV4R269C(high) raised on food with either DMSO or 100 μM GSK219.gSholl analysis of dendritic phenotypes inf. Control fromdshown for reference. Mean ± SEM.n= 6 cells from three larvae for DMSO,n= 10 cells from five larvae for GSK219. Asterisks denote differences from DMSO. Two-way ANOVA (p< 0.0001), Tukey’s post hoc test. Scale bar, 25 µm inaandeand 50 µm incandf. For all panels: *p< 0.05, **p< 0.01, ***p< 0.001, and ****p< 0.0001. To assess mitochondrial axon transport dynamics, we imaged the proximal axon of C4da neurons co-expressing TRPV4(mod) variants and the mitochondrial reporter mito-GFP. We used the TRPV4 R269C (mod) line as it does not exhibit observable morphological phenotypes in C4da neuron axons or their central projections (Supplementary Fig. 3d, e ). TRPV4 R269C (mod) expression significantly inhibits mitochondrial axon transport compared with controls expressing no TRPV4, whereas TRPV4 WT (mod) and TRPV4 R269C+M680K (mod) has minimal impact. Specifically, both anterograde and retrograde axonal mitochondria are more often stationary (Fig. 6a, c ), and retrograde more than anterograde mitochondria have shorter run lengths (Fig. 6d, e ). Fig. 6: Mitochondrial axonal transport is disrupted by TRPV4 R269C prior to axonal degeneration. a Kymographs of mito-GFP transport in the proximal axon of C4da neurons expressing the indicated TRPV4(mod) variants. Scale bar, 10 μm. Quantification of b anterograde duty cycle and c retrograde duty cycle. For control, TRPV4 WT , TRPV4 R269C , TRPV4 R269C+M680K n = 10, 10, 9, 8 and 7, 11, 7, 5 larvae for anterograde and retrograde, respectively. Mean ± SEM. Two-way ANOVA ( p < 0.0001), Tukey’s post hoc test. Frequency distributions of d anterograde and e retrograde mitochondrial run lengths. For control, TRPV4 WT , TRPV4 R269C , TRPV4 R269C+M680K : n = 12, 11 , 14, and 10 larvae; 138, 108, 77, and 72 anterograde and 63, 86, 30, and 29 retrograde runs, respectively. For all panels: * p < 0.05, ** p < 0.01, *** p < 0.001, **** p < 0.0001. 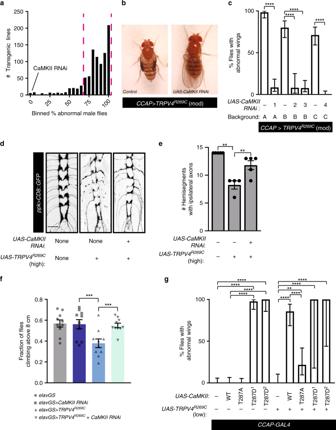Fig. 3: CaMKII is required for TRPV4R269C-mediated neuronal toxicity. aHistogram of results from genetic modifier screen against TRPV4R269Ctoxicity in NCCAP. Dashed magenta lines denote upper and lower bounds of control lines.bImages of flies expressing TRPV4R269C(mod) ± CaMKII RNAi.cPercentage ± 95% CI of flies with unexpanded wings when co-expressing TRPV4R269C(mod) and different CaMKII RNAi fly lines. A = TRiP collection lines, B = Vienna GD collection lines, and C = Vienna KK collection lines. From left to rightn= 65, 59, 60, 25, 65, 66, and 90 flies.Χ2test of all groups (p< 0.0001) followed by pairwise two-sided Fisher’s exact test.dConfocal stacks of axonal projections in C4da neurons expressing TRPV4R269C(high) ± CaMKII RNAi.eMean ± SEM innervation ind.n= 5, 4, and 5 larvae, respectively. One-way ANOVA (p< 0.0002), Tukey’s post hoc test. Scale bar, 25 µm.fClimbing performance of flies 7 days after induction of expression of TRPV4R269C(high) ± CaMKII RNAi with 200 μM RU486. Mean ± SEM.n= 10 vials of 10 flies per genotype. Two-way ANOVA (p< 0.0001), Tukey’s post hoc test.gPercentage ± 95% CI of flies with unexpanded wings when co-expressing TRPV4R269C(low) with variants of CaMKII. T287D1and T287D2denote independentUAS-CaMKIIT287Dlines. From left to rightn= 63, 55, 68, 44, 23, 33, 28, 23, 2, and 3 flies.Χ2test of all groups (p< 0.0001) followed by pairwise two-sided Fisher’s exact test. For all panels: **p< 0.01, ****p< 0.0001. Full size image To test whether pharmacologic activation of TRPV4 WT is sufficient to disrupt mitochondrial transport dynamics, TRPV4 WT (mod) larvae were treated with GSK101. This results in an increased proportion of stationary mitochondria and reduced run length similar to that observed in animals expressing TRPV4 R269C (mod) alone (Fig. 7a, b , Supplementary Fig. 11a, b and d, e). Interestingly, larvae expressing TRPV4 R269C exhibit minimal further disruption of mitochondrial transport in response to GSK101 (Supplementary Fig. 11c, f ), possibly owing to saturation of the molecular machinery responsible for inhibiting transport. We also tested whether treating TRPV4 R269C (mod)-expressing larvae with the TRPV4-selective antagonist GSK219 can ameliorate mitochondrial transport defects. GSK219 normalizes the proportion of motile mitochondria (Fig. 7c, d ) and causes a shift to longer retrograde run lengths in TRPV4 R269C -expressing larvae, but not control larvae (Supplementary Fig. 11g–j ). These data indicate that TRPV4 activation, induced either by the R269C mutation or by a pharmacological agonist, disrupts mitochondrial axon transport. Fig. 7: Pharmacologic manipulation of TRPV4 modulates mitochondrial transport and the mitochondrial transport protein Miro enhances TRPV4 R269C -mediated toxicity. a Kymographs of mito-GFP transport in C4da neuron proximal axons in larvae expressing no TRPV4, TRPV4, or TRPV4 R269C treated with 40 nM GSK101 or DMSO. Scale bar, 10 μm. b Fraction of stationary, anterograde-, and retrograde-moving mitochondria from a . Mean ±SEM. For control, TRPV4 WT , and TRPV4 R269C : DMSO n = 9, 10, 10 larvae; GSK101 n = 10, 14, 11 larvae. Two-way ANOVA ( p < 0.0001), Tukey’s post hoc test. c Kymographs of mito-GFP transport in C4da neuron axons in larvae expressing no TRPV4 or TRPV4 R269C raised on food containing DMSO or 100 µM GSK219 and treated with 10 µM GSK219 during imaging. Scale bar, 10 μm. d Percentage of stationary, anterograde-, and retrograde-moving mitochondria from c . Mean ± SEM. For control and TRPV4 R269C : DMSO n = 11 and 12 larvae; GSK219 n = 14 and 13. Two-way ANOVA ( p < 0.0001), Tukey’s post hoc test. e Percentage ± 95% CI of flies with unexpanded wings when expressing Miro variants ± TRPV4 R269C (low) in N CCAP . From left to right n = 86, 72, 64, 77, 62, 54, 33, 38, 32, 39, 35, and 41 flies. Χ 2 test ( p < 0.0001) followed by pairwise two-sided Fisher’s exact test. f Representative confocal images of C4da neuron projections in larvae expressing TRPV4 R269C (mod) (as in Supplementary Fig. 2d and e) ± overexpressed Miro variants. Similar results observed in all imaged larvae within each genotype ( n = 7, 8, 8, 8, 7, 8, and 8 larvae from left to right) Scale bar, 25 μm. For all panels: * p < 0.05, ** p < 0.01, *** p < 0.001, **** p < 0.0001. Full size image Miro modifies TRPV4 R269C -mediated toxicity Notably, the TRPV4-mediated axonal mitochondrial transport phenotypes (Figs. 6 , 7a–b ) are similar to those seen in Drosophila larvae with homozygous loss-of-function mutations of mitochondrial Rho (Miro) [39] , [40] . Miro is a Ca 2+ -binding GTPase that localizes to the outer membrane of mitochondria and regulates mitochondrial coupling to microtubule motors [38] , [41] , [42] . Miro binds Ca 2+ via two EF hand domains, and this Ca 2+ binding promotes the dissociation of mitochondria from the microtubule motor or microtubule. The amino-terminal GTPase domain of Miro is required for appropriate transport of mitochondria along axons [39] , [40] , [43] , though the specific function of this domain remains unknown. To test whether Miro and TRPV4 function in a common pathway, we tested for genetic interactions between TRPV4 R269C and Miro variants in N CCAP and C4da neurons. While TRPV4 R269C (low) or wild type Miro do not cause a wing phenotype when expressed individually, co-expression of both Miro and TRPV4 R269C (low) cause an ~40% penetrant wing phenotype (Fig. 7e ). Interestingly, expression of a GTP-bound Miro mutant (Miro A20V ) alone is sufficient to cause impaired wing expansion, and this phenotype is not enhanced by co-expression of TRPV4 R269C (Fig. 7e ). Similarly, co-expression of Miro WT or Miro A20V together with TRPV4 R269C (mod) causes axonal degeneration in C4da neurons (Fig. 7f ). Overexpression of Miro WT alone only mildly alters C4da neuron central projections, whereas Miro A20V alone is sufficient to cause axonal degeneration (Supplementary Fig. 12a ). In contrast, expression of a Miro variant locked in the GDP-bound confirmation (Miro T25N ) suppresses the TRPV4 R269C (mod)-mediated wing phenotype and does not cause N CCAP toxicity when co-expressed with TRPV4 R269C (low) (Supplementary Fig. 12b ). In addition, expression of Miro T25N suppresses axonal degeneration in C4da neurons induced by TRPV4 R269C (high) and does not cause toxicity in C4da neurons when co-expressed with TRPV4 R269C (mod) (Supplementary Fig. 12c–d ). These data suggest that GTP binding of the amino-terminal GTPase domain of Miro is necessary and sufficient to promote neurotoxicity downstream of TRPV4 activation. Notably, these genetic interactions are not observed in N CCAP with Miro variants unable to bind Ca 2+ (Miro E234K or Miro E234K+E354K ) (Fig. 7e ). Moreover, Miro variants that cannot bind Ca 2+ do not induce C4da axonal degeneration when co-expressed with TRPV4 R269C (mod) (Fig. 7f ). Thus, Miro-mediated enhancement of TRPV4 R269C -dependent axonal degeneration is dependent on the ability of Miro to bind Ca 2+ , suggesting that TRPV4 R269C causes axonal degeneration by promoting the binding of Ca 2+ to Miro. Inherited motor and sensory peripheral neuropathy, also known as CMT, is the most common form of genetically determined neuromuscular disease [21] . Despite the identification of over 100 causative genes, treatment remains elusive. TRPV4 is one of the rare ion channels that can directly cause peripheral nerve degeneration [1] , [2] , [3] , yet the mechanisms leading to neuronal dysfunction are unknown. In this study, we demonstrate in Drosophila and primary mammalian neurons that a neuropathy-causing mutant, TRPV4 R269C , causes neurodegeneration and increases intraneuronal Ca 2+ via a mechanism that requires a functional ion channel pore (Supplementary Fig. 13). In a genetic screen, we identified CaMKII, a Ca 2+ -dependent kinase, as a potent modifier of TRPV4 R269C -mediated neurotoxicity, unveiling an important role for CaMKII in neuronal TRPV4-associated Ca 2+ signaling. Futhermore, we show that impaired mitochondrial trafficking and the Ca 2+ -binding protein Miro are important determinants of neurotoxicity downstream of TRPV4 activity. Dominant missense mutations in TRPV4 cause a spectrum of in vivo neuropathies that can present congenitally or late in adulthood [1] , [2] , [3] . In this study, we observed cell-autonomous neuronal dysfunction and/or degeneration in multiple Drosophila neuronal subtypes as a consequence of expressing a neuropathogenic mutant form of TRPV4. These phenotypes manifest as early as late larval developmental stages, when abnormalities in neuronal development or maintenance may be relevant, but we also demonstrate that mutant TRPV4 expression can cause adult onset, progressive neuronal dysfunction. Phenotype severity is dependent on TRPV4 expression levels, suggesting that variations in the timing and/or level of TRPV4 expression may be relevant determinants of the marked disease heterogeneity observed in patients. Neuronal dysfunction and degeneration caused by neuropathogenic TRPV4 mutants in vivo were dependent on a functional channel pore, consistent with a gain-of-function mechanism of toxicity. These observations are consistent with prior data in cultured cell lines [1] , [2] , [5] , [6] and the lack of neurodegenerative phenotypes in Trpv4 -null mice [44] , [45] . Furthermore, small molecule inhibition of TRPV4 ameliorates TRPV4-mediated phentoypes in Drosophila , suggesting that TRPV4 antagonism is a promising therapeutic strategy for the treatment of patients with TRPV4-associated neuropathies. TRPV4 inhibition has also been shown to be protective in rodent models of chemotherapy-induced peripheral neuropathy [46] , [47] , suggesting that TRPV4 antagonists may have utility in peripheral neuropathies of diverse etiologies. This is particularly exciting as small molecule TRPV4 antagonists have already proven to be safe in clinical trials for pulmonary edema in heart failure [7] . Our study highlights that increased intracellular Ca 2+ is a fundamental consequence of TRPV4 R269C activation in Drosophila neurons in vivo and in mammalian neurons in vitro. Tightly regulated Ca 2+ homeostasis is critical to myriad aspects of normal neuronal physiology and may be disrupted during neurodegeneration. To identify specific pathways acting downstream of TRPV4 R269C , we conducted, to our knowledge, the largest genetic modifier screen in a Drosophila model of CMT and identified CaMKII as the most potent modifier. We further demonstrated that inhibition of CaMKII ameliorates multiple mutant TRPV4-mediated neuronal phenotypes in flies and also dramatically suppresses TRPV4-mediated intracellular Ca 2+ responses in mammalian neurons. CaMKII is a critical Ca 2+ -sensitive kinase that transduces changes in intracellular Ca 2+ to regulate diverse neuronal processes, including neurite morphogenesis, neuronal excitability, synaptic plasticity, and ion channel activity [28] , [48] . We envision two possible mechanisms by which CaMKII influences TRPV4-mediated increases in intracellular Ca 2+ . First, CaMKII could directly modulate TRPV4 channel gating. Indeed, the gating properties of ion channels such as AMPA receptors can be strongly modulated by CaMKII-dependent phosphorylation [49] . CaMKII is a putative binding partner of TRPV4 [50] , [51] , consistent with the possibility that TRPV4 is directly regulated by CaMKII, but, to our knowledge, no CaMKII-dependent phosphorylation sites in TRPV4 have been identified. A second potential mechanism is that activation of CaMKII by TRPV4-mediated Ca 2+ influx could regulate subsequent TRPV4-independent Ca 2+ release, either by opening of Ca 2+ -permeable channels within the plasma membrane or by activating release of intracellular Ca 2+ stores. Several studies suggest that TRPV4 stimulation orchestrates activation of Ca 2+ -sensitive plasma membrane channels that amplify and propagate Ca 2+ signaling events, and some of these responses can be modulated by inhibition of CaMKII [52] , [53] , [54] , [55] , [56] , [57] . In addition, TRPV4-mediated intracellular Ca 2+ responses can be blunted by depleting endoplasmic reticulum (ER) Ca 2+ stores or by inhibiting ER Ca 2+ release channels, suggesting amplification of signaling by Ca 2+ -mediated ER Ca 2+ release [58] , [59] , [60] . CaMKII can phosphorylate and regulate mammalian IP 3 receptors and ryanodine receptors [61] potentially linking activation of CaMKII with downstream ER Ca 2+ release. Notably, our secondary genetic screen found partial suppression of the wing expansion phenotype with RNAi targeting the Drosophila ryanodine receptor (RyR) (Supplementary Data 2 ). Regardless of the mechanism by which CaMKII influences TRPV4-mediated intracellular Ca 2+ elevations, our results highlight CaMKII as a potent modifier of TRPV4-mediated Ca 2+ signaling and toxicity and add to the growing body of evidence underscoring key roles for CaMKII in neuronal Ca 2+ homeostasis and degeneration [62] , [63] , [64] . Transport of mitochondria within axons is a Ca 2+ -regulated process that is crucial to neuronal homeostasis. Disrupted mitochondrial transport is a common feature across many neurodegenerative diseases, although whether such disruption is an early pathogenic process or a reflection of non-specific neuronal dysfunction is unclear [11] , [12] . In this study, we observed mitochondrial transport defects downstream of neuropathogenic TRPV4 activity prior to the onset of observable degeneration, suggesting that mitochondrial transport impairments are an early pathological event. In addition, mitochondrial transport is impaired by acute activation of TRPV4 WT , demonstrating a close temporal association between TRPV4 activation and impaired mitochondrial transport. As increased intracellular Ca 2+ is sufficient to inhibit the axonal transport of mitochondria [38] , our data are consistent with a model in which TRPV4-mediated Ca 2+ influx serves to regulate the function of axonal mitochondrial transport machinery. In animal models of chemotherapy-induced neuropathy, in which mitochondrial trafficking defects are well-established, inhibition of TRPV4 activity is partially protective [46] , [47] . Our results suggest that blocking TRPV4-mediated disruption of mitochondrial transport may be the mechanism for this protective effect. Our data highlight the importance of the mitochondrial GTPase Miro, which regulates mitochondrial transport in fly and mammalian neurons via mechanisms that rely on the Ca 2+ -binding EF hand domains and amino-terminal GTPase domain, and suggest that Miro provides the link between TRPV4-mediated Ca 2+ elevations and disrupted mitochondrial transport [38] , [39] , [40] , [43] . We observe a marked enhancement of TRPV4 R269C -mediated neurotoxicity by overexpression of wild type Miro, but not by Miro that is unable to bind Ca 2+ , and the GTP-bound form of Miro recapitulates both the wing-opening failure and sensory neuron degenerative phenotypes, independent of TRPV4 expression. Together, these results suggest that dysregulation of Miro is a fundamental downstream effect of TRPV4 activation, as Miro disruption is both necessary and sufficient for the neuronal phenotypes we observe in our TRPV4 fly model. These results are in agreement with prior work highlighting the critical importance of Miro for neuronal health and survival. miro -null flies exhibit severe mitochondrial axon transport defects and early lethality [39] , whereas Miro1 -null mice have degenerative motor neuron disease [65] . Our results linking mitochondrial trafficking impairment and neuronal degeneration closely parallel findings in animal models harboring MFN2 mutations that cause CMT2A. Similar to Miro, MFN2 has myriad roles in mitochondrial biology, and pathogenic MFN2 mutations result in defective mitochondrial fusion and transport [14] , [15] , [66] . MFN2 agonists restore mitochondrial trafficking defects in pre-clinical models of CMT2A [67] , thus establishing a precedent for correcting defects similar to those reported in this study through small molecule manipulation of a mitochondrial GTPase. Moreover, a recent study suggests that CMT2 mutations in both MFN2 and TRPV4 prolong inter-mitochondrial contacts [68] . Further investigation of functional interactions between TRPV4 and mitochondrial biology will help elucidate the precise contributions of these potential pathological mechanisms and could refine therapeutic strategies for a range of neuropathies. In summary, our data support a model in which neuropathogenic TRPV4 mutants cause cell-autonomous neurotoxicity through a gain-of-TRPV4 ion channel function. This results in a CaMKII-dependent increase in neuronal Ca 2+ that disrupts mitochondrial transport and causes axonal degeneration (Supplementary Fig. 13 ). These phenotypes are prevented by TRPV4 antagonists, which hold promise as a therapeutic strategy for the treatment of patients with TRPV4-associated neuropathies. Drosophila stocks and husbandry Flies were raised on a standard cornmeal-molasses food. All experiments were performed at 25 °C with a 12 hour/12 hour day/night cycle, unless otherwise noted. The following stocks were obtained from the Bloomington Stock Center: UAS-CD8::GFP, UAS-mito-GFP, ppk-GAL4, CCAP-GAL4, UAS-GCaMP6s, UAS-miro, UAS-CaMKII RNAi, UAS-CaMKII, UAS-CaMKII T287D , and UAS-CaMKII T287A . UAS-CaMKII RNAi lines (38940, 47280, and 100265) were also obtained from the Vienna Drosophila Research Center. UAS-miro T25N , UAS-miro A20V , UAS-miro E234K , and UAS-miro E234K, E354K were kind gifts from Konrad Zinsmaier. Generation of human TRPV4-expressing Drosophila stocks The human TRPV4 open reading frame (ORF) was PCR amplified from full-length human TRPV4 cDNA in pcDNA3.1 (WT, R269C, R269C + M680K, R232C) [1] using primers (GGGGACAAGTTTGTACAAAAAAGCAGGCTTCACCATGGCGGATTCCAGCGAAGGC and GGGGACCACTTTGTACAAGAAAGCTGGGTCCTAGAGCGGGGCGTCATCAGTCCTCCA) and recombined into pDONR 221 using BP Clonase (Thermo Fisher Scientific). The TRPV4 ORF flanked by attL sites in the resultant entry vectors was fully sequenced and then recombined with either pBID [29] or pTW vectors ( Drosophila Gateway Vector Collection, Carnegie Institution for Science) using LR Clonase (Thermo Fisher). TRPV4(low) lines were generated by microinjection of pBID-UASC-hTRPV4 into M{vas-int.Dm}ZH-2A, y[1]; P{y[+]=CaryP}attP2 embryos by BestGene for PhiC31 site-specific integration at the attP2 site. TRPV4(mod) and TRPV4(high) transgenic lines were microinjected into w1118 embryos for random P -element insertion. Transgenic lines were identified and genetic elements mapped using conventional methods. TRPV4 mRNA and protein expression levels in each transgenic line were determined by reverse transcription quantitative PCR (RT-qPCR) and western blot analyses, respectively (see Methods below). Wing expansion assay Flies carrying the TRPV4 transgene or controls were crossed to w 1118 ; CCAP-GAL4 /TM6B. Flies were transferred to new vials every 3–4 days. After two transfers, the P 0 flies were discarded. Progeny were scored at two times from each vial: 2 and 4 days post eclosion of the first progeny from the cross to eclose. We selected flies carrying the CCAP-GAL4 driver and transgene of interest and scored their wing phenotype by eye using a stereomicroscope. Flies wings were scored as fully expanded, partially expanded, or fully unexpanded. For analysis, partially expanded flies were counted as 0.5 normal and 0.5 unexpanded. Flies that had phenotypic traits of virgins at the time of initial collection were set aside and scored at least 4 hours later. TRPV4 R269C genetic modifier screen Flies of the genotype w 1118 ; CCAP-GAL4 , UAS-TRPV4 R269C (mod) / TM6B, GAL80 were crossed to fly lines containing transposable elements designed to either knockdown or overexpress endogenous Drosophila genes downstream of the GAL4-binding UAS site (Supplementary Data 1 and 2 ). Putative modifier genes were selected based on their potential to be druggable [27] , CMT genes, and other genes implicated in TRPV4 signaling. We selected for flies carrying CCAP -GAL4, UAS - TRPV4 R269C , and the screen element and scored their wing phenotypes as described above. For experiments studying genetic interactions with TRPV4 R269C (low), flies of the genotype w 1118 ; CCAP-GAL4/ CyO; UAS-TRPV4 r269C (low)/TM6B were used. Climbing assays We crossed our transgenic TRPV4(high) lines to flies carrying the elav-GeneSwitch driver. P 0 flies were transferred to new vials every 3–4 days and were discarded after the second transfer. Progeny were allowed to develop on standard food. Upon eclosion, we selected flies carrying TRPV4 transgenes and the elav-GeneSwitch driver. Zero- to 3-day old flies were then transferred onto food containing 200 μM RU486 (Sigma) at a density of 10 flies per vial. Flies were transferred onto fresh RU486 food every 2 days. Climbing behavior was scored by transferring flies into a climbing assay chamber which was composed of two vials without food stacked on top of one another such that the two openings faced one another. Lines were drawn on the vials 8 cm from either end. Once flies were in the vial, the vial was tapped swiftly four times on the laboratory bench so as to knock all flies to the bottom. Flies were then allowed to climb for 10 seconds at which point we counted the number of flies above and below the 8 cm line. Flies were allowed to rest for 1 minute and the process was repeated for a total of 10 trials per vial of 10 flies. RT-qPCR and western blot analyses Analyses of TRPV4 mRNA and protein levels were performed utilizing adult flies expressing TRPV4 variants selectively in neurons ( C155 - GAL4 pan-neuronal driver). Heads were collected from adult flies at 1–3 days post eclosion and stored at −80 °C. For quantification of TRPV4 transcript levels, heads were homogenized in Trizol (ThermoFisher) using plastic pestles and RNA isolated using the RNeasy mini kit (Qiagen) including on-column DNase digestion. Following cDNA conversion utilizing the High Capacity cDNA Reverse Transcription kit (ThermoFisher), RT-qPCR was performed with the HT7900 Real-Time PCR system (ThermoFisher) using Taqman Universal PCR master mix and the following Taqman assays: human TRPV4 exons 3–4 (Hs01099348_m1), human TRPV4 exons 5–6 (Hs00540967_m1), human TRPV4 exons 7–8 (Hs00222101_m1), Drosophila RpII140 (Dm02134593_g1; all from ThermoFisher). For western blot analyses, samples were lysed in RIPA buffer (Sigma) supplemented with protease inhibitors (Cell Signaling Technology) and sonicated. Protein lysates were resolved on 4–15% TGX gels (Bio-Rad) and transferred to PVDF membranes (ThermoFisher). Primary antibodies used were polyclonal rabbit anti-TRPV4 (1:500; Abcam; ab39260), monoclonal rabbit anti-β-actin (1:1000; Cell Signaling Technology; #4970), and monoclonal mouse anti-GAPDH (1:5000; ThermoFisher; #AM4300), followed by HRP-conjugated mouse anti-rabbit (1:150,000; Jackson ImmunoResearch; #211-032-171) or goat anti-mouse (1:150,000; Jackson ImmunoResearch; #211-032-171) secondary antibodies. Membranes were developed using SuperSignal West Femto Maximum Sensitivity Substrate (ThermoFisher) and imaged using an ImageQuant LAS 4000 system (GE Healthcare). Larval dissections and immunostaining Larvae were filleted in HL3 solution to expose the CNS and body wall, prior to fixation in 4% paraformaldehyde (PFA) in PBS for 20 minutes at room temperature with gentle shaking. Preparations were then washed three times over 10 minutes in PBS and blocked for 1 hour at room temperature in 5% normal goat serum in PBS with 0.1% Triton X-100 (PBST). Fillets were then incubated with primary antibody for 2 hours at room temperature or overnight at 4 °C in 5% normal goat serum in PBST. 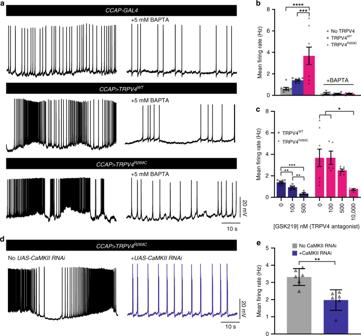Fig. 4: TRPV4R269Cmediates a reversible, Ca2+- and CaMKII-dependent increase in neuronal excitability. aTraces of NCCAPspontaneous activity in flies expressing no TRPV4, TRPV4WT(mod), or TRPV4R269C(mod) ± 5 mM BAPTA.bMean firing rates froma. Mean ± SEM.n= 9 (no TRPV4), 8 (TRPV4WT), 9 (TRPV4R269C), 5 (no TRPV4 + BAPTA), 5 (TRPV4WT+ BAPTA), and 6 (TRPV4R269C+ BAPTA) flies. Two-way ANOVA (p= 0.0017), Tukey’s post hoc test.cMean firing rate after incubation with GSK219. Mean ± SEM. TRPV4WTn= 8, 6, and 4 flies for 0, 100, and 500 nM TRPV4R269Cn= 8, 5, 8, and 4 flies for 0, 100, 500, and 10,000 nM. 0 nM values are the same as shown inb. One-way ANOVA (p< 0.0001 (TRPV4WT),p= 0.0169 (TRPV4R269C)), Tukey’s post hoc test.dTraces of NCCAPspontaneous activity in flies expressing TRPV4R269C± CaMKII RNAi.eMean firing rate ind. Mean ± SEM.n= 6 per genotype. Unpaired two-tailedttest.p= 0.0017. For all panels: *p< 0.05, **p< 0.01, ***p< 0.001, ****p< 0.0001. Primary antibodies included mouse anti-GFP IgG2a (1:1000, ThermoFisher, A-11120) and rabbit anti-GFP (1:1000, ThermoFisher, A-11122). They were then washed three times over the course of 1 hour with PBST and were then incubated for 1 hour with secondary antibody in 5% normal goat serum in PBST. Secondary antibodies included DyLight 488-conjugated goat anti-mouse IgG2a (1:1000, Jackson ImmunoResearch, 115-285-206) and Alexa Fluor 488-conjugated goat anti-rabbit IgG (1:1000, ThermoFisher, A-11034). Fillets were then mounted onto glass slides in Fluoromount-G (Southern Biotech) or Vectashield (Vector Labs) mounting media. Ca 2+ imaging in Drosophila dendritic arborization neurons 120 h AEL third instar larvae expressing GCaMP6s were pinned ventral side up on silicone elastomer plates and dissected in external saline solution composed of: NaCl 120 mM, KCl 3 mM, MgCl 2 4 mM, CaCl 2 1.5 mM, NaHCO 3 10 mM, trehalose 10 mM, glucose 10 mM, TES 5 mM, sucrose 10 mM, and HEPES 10 mM. 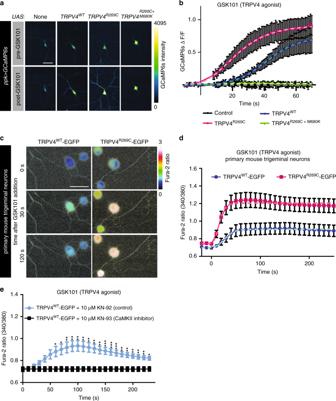Fig. 5: The R269C mutation enhances TRPV4-mediated Ca2+influx in fly and mouse neurons. aConfocal images of GCaMP6s in larval C4da neurons expressing the indicated transgenes before and 180 s after application of 40 nM GSK101 att= 0 s. Scale bar, 50 μm.bChange in somal GCaMP6s fluorescence over baseline (ΔF/F) of the genotypes shown ina. Mean ± SEM.n= 8 (no TRPV4), 8 (TRPV4WT), 7 (TRPV4R269C) and 10 (TRPV4R269C+M680K). Non-linear regression (dashed lines, logistic model) indicates TRPV4WTt1/2max= 41 ± 3.0 s was greater than TRPV4R269Ct1/2max= 22 ± 2.4 s (p< 0.0001, unpaired two-tailedttest). Maximum response 0.91 (TRPV4R269C) and 0.73 (TRPV4WT) (p= 0.06, unpaired two-tailedttest)cImages of the Fura-2AM ratio in primary mouse trigeminal neurons transduced with TRPV4WTor TRPV4R269Cbefore and after the application of 30 nM GSK101. Scale bar, 50 μm.dMean ± SEM Fura-2AM ratio over time of the images inc. Drug added att= 0.n= 44 (TRPV4WT) and 48 (TRPV4R269C) neurons from 12 wells per genotype from three separate preparations. Non-linear regression (dashed lines, logistic model) indicates TRPV4WTt1/2max= 28 ± 8.5 s and TRPV4R269Ct1/2max= 16 ± 3.8 s (p= 0.2, unpaired two-tailedttest). Maximum responses TRPV4WT= 0.9, TRPV4R269C= 1.2 (p< 0.0001, unpaired two-tailedttest).eMean ± SEM Fura-2AM ratio over time in response to 30 nM GSK101 att= 0 in neurons expressing TRPV4WTand pre-treated for 4 hours with 10 μM KN-93 or KN-92,n= 44 (KN-92) and 28 neurons (KN-93) from 12 wells per genotype from three separate preparations. Two-way ANOVA, Geisser-Greenhouse correction (p< 0.0001), Tukey’s post hoc test. For all panels: *p< 0.05,**p< 0.01, ***p< 0.001. The osmolality was 305 mOsm kg −1 , and the pH was 7.25. Internal debris was removed with forceps and the body wall pinned flat. Time-lapse imaging was performed under a water-immersion objective lens (W Plan-Apochromat ×20/1.0 DIC CG = 0.17 M27 75 mm) using a Zeiss LSM-700 confocal microscope. Frame rate was 1.27 Hz. Regions of interest (ROIs) were drawn around entire somata for trace examples. 5 µm diameter circle ROIs were placed on brightest part of each soma to calculate responses to 40 nM GSK101 or DMSO, which were added directly to the recording media. Imaging of sponataneous calcium transients with GCaMP5-myr was performed on a Zeiss Axio-Observer widefield micrscope using a ×63 oil immersion lense. Larvae were dissected ventral side down in HL3 with 2.0 mM Ca 2+ on a sylgard block. After removal of the internal tissues, the sylgard block to which the fillet was pinned was inverted and placed down on a large, circular glass coverslip such that the fillet rested against the coverslip while immersed in HL3. Images were acquired at a rate of four frames per second for one minute with excitation from a 475 nm LED light source. The acquired image series were then blinded, and an experimenter who was not involved in image acquisition counted the number of calcium transients, defined as clear, observable increases in GCaMP5-myr fluorescence intensity throughout each movie. Mouse husbandry All mice used in this study were housed and handled according to protocols approved by the Animal Care and Use Committee of Johns Hopkins University School of Medicine. Mouse trigeminal neuron isolation and culture Six to 10 week-old C57BL/6 J mice were deeply anesthetized with isoflurane and killed by cervical dislocation. The bilateral trigeminal ganglia were then harvested and dissociated via consecutive incubations in Hibernate (Brain Bits) with papain (37 °C 20 min, gentle agitation at 10 min) followed by collagenase/dispase (37 °C 20 min, gentle agitation at 10 min) [69] . After enzyme incubations, harvested ganglia were gently titruated 2–3 time with a P1000 pipette tip followed by an additional 2–3 passes through a P200 pipette tip. Titurated ganglia were carefully overlayed on a Percoll gradient and centrifuged at 1500 × g for 20 min. The top layer was carefully removed and centrifuged for 10 min at 1000 × g. Trigeminal neurons were plated on poly- l -ornithine and collagen/laminin coated eight-well Borosilicate coverglass imaging chambers (ThermoFisher). Neurons were transduced with virus carrying GFP, TRPV4 WT -EGFP, or TRPV4 R269C -EGFP 24 hours after plating. Experiments were performed 72 hours after viral transduction. Lentivirus production TRPV4 WT and TRPV4 R269C with a C-terminal EGFP tag in pcDNA3.1 were subcloned into the lentivirus transfer vector FUGW (gift from David Baltimore, Addgene plasmid #14883) (PMID 11786607). In brief, TRPV4-EGFP was PCR amplified (Forward primer: CTTGGGCTGCAGGTCGACTCTAGAGATGGCGGATTCCAGCGAAG, Reverse primer: TTGATTATCGATAAGCTTGATATCGTTACTTGTACAGCTCGTCCATG) and subcloned into the EcoRI and BamHI restriction sites of the FUGW plasmid using the Gibson Assembly Cloning Kit (New England Biolabs). Lentivirus was produced by transfecting HEK293T cells with second generation packaging vectors pCMV-VSV-G and pCMV-dR8.91 (gifts from Jeffrey Rothstein) along with FUGW TRPV4-EGFP (WT or R269C). HEK293T cells were transfected using polyethylenimine (PEI) and virus-containing media was harvested at 48 and 72 hours post transfection and concentrated using Lenti-X Concentrator (Takara). Trigeminal neuron Ca 2+ imaging Virally transduced trigeminal neurons and 50B11 cells were loaded with the ratiometric Ca 2+ indicator Fura-2AM (ThermoFisher) for 1 hour at 37 °C per the manufacturer’s instructions. Ca 2+ imaging was performed on a Zeiss AxioObserver.Z1 inverted microscope equipped with a Lambda DG-4 (Sutter Instrument Company) wavelength switcher. Prior to Ca 2+ imaging of trigeminal neurons, a single channel GFP image was acquired to measure TRPV4 expression within individual neurons. Cells were imaged at 340 nm and 380 nm excitation at three 10 second intervals to acquire a baseline fluorescence measurement prior to the application of the TRPV4-selective agonist GSK1016790A (MilliporeSigma), after which cells were imaged for ~4 minutes at a rate of one frame per 10 seconds. Baseline calcium was determined at t = −10 s, the timepoint immediately prior to addition of GSK1016790A. The CaMKII inhibitor KN-93 and its inactive analog KN-92 (Cayman Chemical) were used at 10 μM and applied for 4 hours prior to imaging. AIP (MilliporeSigma) was used at 10 μM and applied two hours prior to imaging. Trigeminal neuron fixation and immunostaining Coverslips with transduced trigeminal neurons were washed three times quickly with PBS. Neurons were then fixed for 15 minutes at room temperature in 4% PFA. PFA was removed and coverslips were rinsed with PBS. Neurons were then permeabilized with PBS plus 0.1% TritonX-100 (PBST) for 10 minutes. Coverslips were then washed briefly with PBS and incubated with mouse anti-GFP IgG2a (1:1000, ThermoFisher, A-11122) and chicken anti-TUJ1 (1:1000) antibodies diluted in blocking buffer (4% normal goat serum in PBST) overnight with gentle shaking at 4 °C. Coverslips were then washed six times, 10 minutes each in PBST and were then incubated with DyLight 488-conjugated goat anti-mouse IgG2a (1:1000, Jackson ImmunoResearch, 115-285-206) and Alexa Fluor 555-conjugated goat anti-chicken (1:1000, ThermoFisher, A-21437) secondary antibodies in blocking buffer for 1 hour at room temperature with gentle shaking. Coverslips were then washed six times, 10 minutes each in PBST. Coverslips were than mounted with VectaShield+DAPI (Vector Labs) and sealed with nail polish. Confocal microscopy-fixed imaging Slides were imaged on a Zeiss 800 LSM confocal laser scanning microscope with a ×20 air, ×40 oil immersion, or ×63 oil immersion objective. Image acquisition parameters were kept uniform across all samples in a given experiment. Confocal microscopy and live imaging of trigeminal neurons Transduced trigeminal neurons were incubated for 2 hours with 10 μM KN-92 or KN-93. Neurons were then incubated for 20 minutes with ER-Tracker Red (0.5 μM, ThermoFisher, E34250) diluted in artificial cerebrospinal fluid (aCSF) with either KN-92 or KN-93. Wells were then washed quickly three times with pre-warmed aCSF, and cells were finally placed in pre-warmed aCSF with either 10 μm KN-92 or 10  μm KN-93. Neurons were imaged on a Zeiss 800 LSM confocal laser scanning microscope with a ×63 Plan-apochromat oil immersion lens. Live cell imaging of axonal transport in Drosophila Mito-GFP was used to label mitochondria and was expressed in C4da neurons along with TRPV4 using the ppk-GAL4 driver. Wandering third instar larvae were dissected in HL3 solution with 0.6 mM Ca 2+ and 4 mM glutamate as described [70] . Larvae were then mounted in HL3 solution on glass slides with the coverslip secured via dental glue (Surgident, #50092189). For experiments involving drug treatments, drug was added to the dissection media and allowed to incubate at least 5 minutes prior to image acquisition. Imaging was performed on a Zeiss 800 LSM with a ×63 oil objective. Image series of C4da neuron axons were captured in a single focal plane at an acquisition rate of 1 frame/second for 2 minutes, in a 200 μm~500 μm window from the cell body in abnominal segements A6 and A7. Movement dynamics were calculated by tracking the position of individual mitochondria frame by frame in ImageJ as previously described [70] . Since one pixel represents 0.198 μm in our image acquisition, only net velocities >0.2 μm/s with more than three consecutive frames in one direction were considered as anterograde or retrograde. Moving mitochondria that could be tracked for >60 frames continuously were considered for measuring mitochondrial run length or duty cycle, and representative kymographs were generated from the acquired time-lapse images using Zeiss Zen Blue 2.3 software. For experiments involving GSK1016790A, larvae were bathed in recording media which contained GSK1016790A during mounting for imaging. For experiments involving GSK2193874, larvae were raised on food with 10 μM GSK2193874 due to the observed insensitivity of TRPV4 R269C to this compound in electrophysiologic recordings (Fig. 4c ). Larvae were also bathed in recording media with 10 μM GSK2193874 during dissection and mounting for imaging. Electrophysiological recordings of N CCAP Experiments were performed on 1–3-day old adult female flies. Perforated patch-clamp recordings with β-escin were performed as previously described with minor modifications [25] , in order to measure action potentials (APs) from CCAP neurons located in the brain. Brains were removed and dissected in a Drosophila physiological saline solution (101 mM NaCl, 3 mM KCl, 1 mM CaCl 2 , 4 mM MgCl 2 , 1.25 mM NaH 2 PO 4 , 20.7 mM NaHCO 3 , and 5 mM glucose; pH 7.2), which was pre-bubbled with 95% O 2 and 5% CO 2 . To better visualize the recording site, the perineuronal sheath surrounding the brain was focally and carefully removed after treating with an enzymatic cocktail, collagenase (0.4 mg/ml) and dispase (0.8 mg/ml), at 22 °C for 1 minute and cleaning with a small stream of saline pressure-ejected from a large diameter pipette using a 1 mL syringe. In addition, prior to recording, cell surfaces were cleaned with saline pressure-ejected from a small diameter pipette, using a 1 ml syringe connected to the pipette holder. The recording chamber was placed on an X–Y stage platform (PP-3185-00; Scientifica, UK). The cell bodies of the targeted CCAP neurons were visualized with CD8:GFP fluorescence on a fixed-stage upright microscope (BX51WI; Olympus, Japan) and viewed with a ×40 water-immersion objective lens (LUMPlanFl, NA: 0.8, Olympus). Patch pipettes (8–12 MΩ) were fashioned from borosilicate glass capillaries without filaments (OD/ID: 1.2/0.68 mm, 627500, A-M systems, WA) using a Flaming-Brown puller (P1000; Sutter Instrument), and further polished with a MF200 microforge (WPI) prior to filling with the internal pipette solution (102 mM potassium gluconate, 0.085 mM CaCl 2 , 0.94 mM EGTA, 8.5 mM HEPES, 4 mM Mg-ATP, 0.5 mM Na-GTP, 17 mM NaCl; pH 7.2). Biocytin hydrazide (13 mM; ThermoFisher) was added to the pipette solution before the recording. Recordings were acquired with an Axopatch 200B amplifier (Molecular Devices) and sampled with a Digidata 1440 A interface (Molecular Devices). These devices were controlled via pCLAMP 10 software (Molecular Devices). The signals were sampled at 20 kHz and low-pass filtered at 2 kHz. Junction potentials were nullified prior to high-resistance (GΩ) seal formation. Cells showing evidence of “mechanical” breakthrough, as assessed by the abrupt generation of a large capacitance transient (as opposed to the more progressive, gradual one generated by chemical perforation) were excluded. One CCAP neuron per brain was recorded. During the recording, the bath solution was slowly but continuously exchanged with fresh saline by means of a gravity-driven system (approximate flow rate of 1–2 ml/min). The mean firing rate of spontaneous APs and RMP were determined by the mean value of voltage during zero-holding current (0 pA as I hold ) gap-free recording. For quantifying intrinsic membrane excitability, APs were elicited in response to current injections with 300 ms stepping pulses at 20 pA increments up to 100 pA. Electrophysiological analysis of both spontaneous APs and evoked APs was performed using custom MATLAB-based software. APs were detected automatically by identification of local maxima and were then manually curated to remove excitatory post-synaptic potentials using minimum voltage threshold criteria. Frequency of detected APs was quantified as mean firing rate during current injection. The current threshold (minimum current to evoke spiking) and the slope of the f–I curve were determined by linear regression of the curve from the point of initial spiking. To analyze subthreshold membrane potential dynamics as Δramp, spontaneous APs were first removed from the raw traces by introducing median filter and smoothing using a 7–18 ms (depending on spike width) moving average. Δramp was then quantified as the difference between the most depolarized value and the most hyperpolarized value during the recording. Internal Ca 2+ chelation experiments were carried out by intracellular perfusion with the Ca 2+ chelator, BAPTA. For experiments with intracellular perfusion of BAPTA, a conventional whole-cell patch technique was used. Patch pipettes filled with internal pipette solution containing 5 mM BAPTA were brought up to the cell bodies. After GΩ seal formation, the patched membrane was ruptured by applying negative pressure. Data acquisitions of membrane potential were initiated 5 min following the rupture of the membrane. GSK2193874 was prepared as a 20 mM stock solution dissolved in DMSO, and this stock was mixed into Drosophila physiological saline solution at a final concentration of 100 nM, 500 nM, or 10 μM. To achieve substantial penetration of the drug into the whole-brain tissue preparation, data acquisitions of membrane potential were carried out after 60 min bath application of the drug as preincubation period. During the preincubation period, 95% O 2 and 5% CO 2 pre-bubbled Drosophila physiological saline solution containing the drug was continuously perfused by Peristaltic pump (MINIPULS 3, Gilson) with flow rate of 2–3 ml/min. Recovery was not tested because of the considerable amount of time required to wash out drugs, in particular hydrophobic compounds, such as GSK2193874. After recording the physiological responses of N CCAP , biocytin hydrazide was iontophoresed into the cell with a constant hyperpolarizing current of 0.9–1.2 nA passed for at least 5 minutes. The brain was then fixed in 4% PFA in PBS overnight at 4 °C. After washing for 1 hour in several changes of PBST (0.3% Triton X-100 in PBS) at room temperature, the brain was incubated with a mouse anti-GFP antibody (Invitrogen, 1:200) for 16-40 hours on a shaker at 4 °C, followed by incubation with an Alexa Fluor 488-conjugated goat anti-mouse (Invitrogen, 1:1000) secondary antibody and Alexa Fluor 568-conjugated streptavidin (Invitrogen, 1:100) for 24–40 hours on a shaker at 4 °C. After a 1 hour wash, samples were cleared in 70% glycerol in PBS for 5 minutes at room temperature and then mounted in Vectashield (Vector Labs). Recorded CCAP neurons were imaged using a confocal imaging system (LSM-700; Carl Zeiss). Image analysis Fluorescent images were analyzed using ImageJ (NIH) or Imaris (Bitplane, Zurich, Switzerland). Synaptic area measurements were acquired in ImageJ using the Analyze Particles tool. In brief, confocal stacks were converted to maximum intensity projections and background fluorescence subtracted using the Math function. The image was then thresholded and an ROI was drawn around the segment to be measured and CD8-GFP positive area was measured using the Analyze Particles tool. Dendritic branching was measured in ImageJ or Imaris. In ImageJ confocal stacks were converted to maximum intensity projections, background fluorescence was then subtracted and the image was thresholded and converted to a binary image. Branching was measured using the Sholl analysis tool. In Imaris, dendrites were semi-automatically traced using the Filaments tool. In brief, images were thresholded to identify the center and seed points, filaments were then manually evaluated and incorrected tracings were removed and missing tracings were added. Branching was assessed using the Sholl branching tool. In either software, the spacing of the Sholl radii was 10 μm. 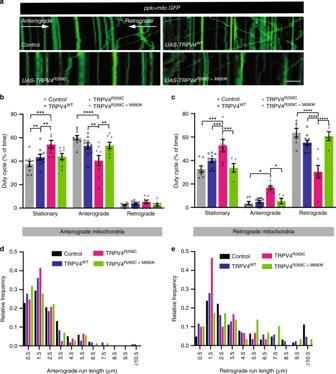Fig. 6: Mitochondrial axonal transport is disrupted by TRPV4R269Cprior to axonal degeneration. aKymographs of mito-GFP transport in the proximal axon of C4da neurons expressing the indicated TRPV4(mod) variants. Scale bar, 10 μm. Quantification ofbanterograde duty cycle andcretrograde duty cycle. For control, TRPV4WT, TRPV4R269C, TRPV4R269C+M680Kn= 10, 10, 9, 8 and 7, 11, 7, 5 larvae for anterograde and retrograde, respectively. Mean ± SEM. Two-way ANOVA (p< 0.0001), Tukey’s post hoc test. Frequency distributions ofdanterograde anderetrograde mitochondrial run lengths. For control, TRPV4WT, TRPV4R269C, TRPV4R269C+M680K:n= 12, 11,14, and 10 larvae; 138, 108, 77, and 72 anterograde and 63, 86, 30, and 29 retrograde runs, respectively. For all panels: *p< 0.05, **p< 0.01, ***p< 0.001, ****p< 0.0001. 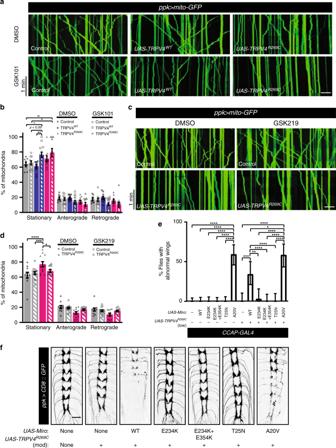Fig. 7: Pharmacologic manipulation of TRPV4 modulates mitochondrial transport and the mitochondrial transport protein Miro enhances TRPV4R269C-mediated toxicity. aKymographs of mito-GFP transport in C4da neuron proximal axons in larvae expressing no TRPV4, TRPV4, or TRPV4R269Ctreated with 40 nM GSK101 or DMSO. Scale bar, 10 μm.bFraction of stationary, anterograde-, and retrograde-moving mitochondria froma. Mean ±SEM. For control, TRPV4WT, and TRPV4R269C: DMSOn= 9, 10, 10 larvae; GSK101n= 10, 14, 11 larvae. Two-way ANOVA (p< 0.0001), Tukey’s post hoc test.cKymographs of mito-GFP transport in C4da neuron axons in larvae expressing no TRPV4 or TRPV4R269Craised on food containing DMSO or 100 µM GSK219 and treated with 10 µM GSK219 during imaging. Scale bar, 10 μm.dPercentage of stationary, anterograde-, and retrograde-moving mitochondria fromc. Mean ± SEM. For control and TRPV4R269C: DMSOn= 11 and 12 larvae; GSK219n= 14 and 13. Two-way ANOVA (p< 0.0001), Tukey’s post hoc test.ePercentage ± 95% CI of flies with unexpanded wings when expressing Miro variants ± TRPV4R269C(low) in NCCAP. From left to rightn= 86, 72, 64, 77, 62, 54, 33, 38, 32, 39, 35, and 41 flies.Χ2test (p< 0.0001) followed by pairwise two-sided Fisher’s exact test.fRepresentative confocal images of C4da neuron projections in larvae expressing TRPV4R269C(mod) (as in Supplementary Fig. 2d and e) ± overexpressed Miro variants. Similar results observed in all imaged larvae within each genotype (n= 7, 8, 8, 8, 7, 8, and 8 larvae from left to right) Scale bar, 25 μm. For all panels: *p< 0.05, **p< 0.01, ***p< 0.001, ****p< 0.0001. Statistical analysis Statistical analyses were performed in Prism 7.0 (GraphPad). For normally distributed datasets comparing summative statistics (e.g., mean) an unpaired t test, or a one- or two-way analysis of variance (ANOVA) was used, as appropriate. For data sets of repeated measures (e.g., calcium imaging over time), a two-way ANOVA with a Geisser-Greenhouse correction was used. If the ANOVA detected a significant interaction ( α = 0.05), Tukey’s post hoc test was performed to identify which groups were significantly different. The level of significance is indicated as * p < 0.05, ** p < 0.01, *** p < 0.001, **** p < 0.0001. Sample sizes (“ n ”) and indicators of statistical significance are noted within the Figure legends. For all graphs of Drosophila wing expansion, data are presented as a percentage of whole. The error bars in those graphs depict the 95% confidence intervals that were calculated using the Wilson/Brown method. A Χ 2 test across all experimental groups was performed to test for the presence of any interaction. Pairwise Fisher’s exact tests were then performed between relevant groups to assess for significant inter-group differences. Reporting summary Further information on research design is available in the Nature Research Reporting Summary linked to this article.